Electron correlations in MnxGa1–xAs as seen by resonant electron spectroscopy and dynamical mean field theory After two decades since the discovery of ferromagnetism in manganese-doped gallium arsenide, its origin is still debated, and many doubts are related to the electronic structure. Here we report an experimental and theoretical study of the valence electron spectrum of manganese-doped gallium arsenide. The experimental data are obtained through the differences between off- and on-resonance photo emission data. The theoretical spectrum is calculated by means of a combination of density-functional theory in the local density approximation and dynamical mean field theory, using exact diagonalization as impurity solver. Theory is found to accurately reproduce measured data and illustrates the importance of correlation effects. Our results demonstrate that the manganese states extend over a broad range of energy, including the top of the valence band, and that no impurity band splits-off from the valence band edge, whereas the induced holes seem located primarily around the manganese impurity. The field of diluted magnetic semiconductors (DMS) [1] , [2] has for the past decade broadened to include several aspects of materials science, for example, materials synthesis in bulk- and thin-film form, structural and magnetic characterization, photo-electron spectroscopy for characterization of the electronic structure and theoretical approaches based on model Hamiltonians or first-principles calculations. Several reviews have lately been authored [3] , [4] , [5] , [6] , [7] , presenting the evolution of the field starting from the first reports on magnetic impurities in semiconductors [8] , [9] . A milestone event was the report on carrier-mediated ferromagnetism of Mn-doped InAs and GaAs [1] , where the Mn atoms both act as acceptors and magnetic impurities. In practical applications of spintronics, an ordering temperature above room temperature is needed, and a few systems were predicted [2] to be promising from that point of view, namely Mn-doped ZnO and Mn-doped GaN. Unfortunately, it has proven very difficult to determine their ordering temperatures experimentally, and values ranging from close to 1,000 K to just above 0 K have been reported. This vast spread of values can possibly be linked to difficulties in synthesizing samples with a homogeneous distribution of substitutional Mn atoms in the host lattice. Mn-doped GaAs offers a considerably more robust situation from a synthesis point of view, and substitutional Mn doping at the Ga sites can reach concentrations up to ~15% (refs 10 , 11 ), as estimated from saturation magnetization data. The magnetic ordering temperature ( T C ) depends on the detailed preparation procedures and evaluation methods [11] , [12] , [13] , the highest reported value being between 188 K (ref. 14 ) and about 200 K (ref. 15 ), inferred, respectively, from the measured magnetization and from the maximum in the resistivity curve (the latter method is known to overestimate the transition temperature [10] ). On the theory side, it has been suggested [2] that the ferromagnetic interaction in Mn-doped GaAs is described by Vonsovsky–Zener’s p–d exchange model [16] , [17] . The main assumptions of this model are that the Mn-3d electrons are localized and that the divalent Mn impurities can induce itinerant spin-carriers (holes) in the valence band of the host material [4] , [18] . These holes couple anti-ferromagnetically to the localized moments and mediate an effective long-range exchange interaction between the moments themselves [2] , [18] . The picture of long-ranged interactions has, however, been challenged by calculations based on first-principles theory, albeit without correlation effects taken into account. These works suggest that the spin-carrying holes are more bound to the Mn impurity and arise from a narrow impurity band of mixed spd character [4] , [6] . As a result, a much more short-ranged interaction is observed, with magnetic percolation as a key ingredient, and a decent agreement is found between calculated and observed ordering temperatures [19] , [20] . This situation is better described by the double-exchange model, which was originally introduced for mixed-valence dense ferromagnets [21] and later on adapted to DMS [4] , [6] , [22] , [23] . In the double-exchange model it is not crucial whether the main character of the carriers is 3d (refs 6 , 7 ) or 4p (refs 4 , 24 ) as this does not affect either the basic physics (dependence of the effective hopping parameter on the magnetic configuration) or the form of the effective magnetic Hamiltonian [25] , [26] . Instead, the essential condition is that the band crossing the Fermi level has a width that is smaller than the effective exchange energy between localized moments and spin-carrying holes [4] . This is opposite to the situation of the aforementioned p-d exchange model, where the exchange energy is smaller than the bandwidth of the carriers. In this view, double-exchange and p-d exchange are both due to the hybridization between conduction and magnetic electrons, and are, respectively, associated to the limit of narrow and broad bands [4] , [22] , [27] . Apart from first-principles studies, a significant contribution from the double-exchange mechanism in Mn-doped GaAs is also suggested in a recent experimental study [28] . Here, an impurity level, which was intersected by the Fermi level, was conferred to lie in the band gap. The experimental work of Dodobrowolska et al . [29] comes to similar conclusions. In particular, it was reported that the Fermi level lies above the top of the valence band, and although a direct measurement of an impurity band was lacking, the authors interpreted their data in terms of the existence of such a feature. Spectroscopic investigations, based on hard X-ray angle-resolved photo-emission [30] , do not find such an impurity level. This work instead proposed that both p-d as well as double exchange are active in Mn-doped GaAs, as suggested in the study by Sato et al . [6] One must conclude that there is a lack of consensus regarding the mechanisms behind magnetism in Mn-doped GaAs and possibly DMS systems in general. The shortcoming in understanding magnetism in these materials is coupled to the lack of a precise knowledge of their electronic structure. A weak point in previous first-principles studies through density-functional theory is that the calculations are based on a mean-field-like description of the electronic structure, using the local density approximation (LDA) or the generalized gradient approximation. The main criticism to this theory is that a mean-field-like description may not be sufficiently accurate for describing the Mn-3d states, and that correlation effects due to the strong Coulomb interaction must be considered [7] . Indeed, calculations including correlation effects have been made for simplified models with reduced degrees of freedom, using several adjustable parameters [31] , [32] , [33] , [34] . Although these models have been important to identify the different competing mechanisms in various parameter regimes, their applicability to Mn-doped GaAs cannot be inferred from a comparison with an accurate experimental photo-emission spectrum. Among the published studies, the only materials-dependent theory including electron–electron interaction directly is the mean-field (static) LDA+U method [6] , [35] , [36] , [37] , [38] ; however, as we show below, this method is inaccurate when it comes to reproducing the measured electronic structure of Mn-doped GaAs. The discussion above indicates that a thorough analysis of the electronic structure of Mn-doped GaAs is highly needed, combining experimental data with accurate theory, to clarify the role of electron correlations and their impact on magnetism. Recent studies regarding the coupling of the electronic structure to the nature of the magnetic interactions [29] , and the resulting debate on their validity [39] , [40] , further highlight this need. The purpose of this article is to provide such an analysis, and we present here the spectral properties of Mn-doped GaAs as given by differences between off- and on-resonance photo-emission data for 0.1, 1 and 6% Mn doping. The experimental results are compared with electronic structure calculations based on a combination of density-functional theory and dynamical mean field theory (LDA+DMFT) [27] , [41] , [42] . Both theory and experiment are focused on the high-temperature paramagnetic phase, as described in the Methods section. Correlated Mn-3d states In Fig. 1 , the experimental data for the Mn-3d excitation spectra are reported for samples with a Mn concentration of 0.1, 1 and 6%. The curves were extracted by taking differences between off- and on-resonance photon energies for the Mn-3d cross-section. In Fig. 2 the experimental spectrum for the sample with 1% Mn concentration is directly compared with the LDA+DMFT projected density of states (PDOS) of the Mn-3d orbitals, for 3.7% Mn concentration. For such concentrations of Mn, the direct wave-function overlap between different Mn atoms is vanishingly small, and it is expected that the spectral properties are rather insensitive to smaller modifications of the Mn concentration (as Fig. 1 also shows). Comparison with the more diluted experimental spectrum is motivated by the fact that at high Mn concentrations the spectrum is broadened due to a statistical (that is, non-uniform) Mn distribution. [43] For Mn atoms occupying Ga sites in the zincblende structure, the probability for finding two nearest neighbour sites occupied is 30% at 3% Mn concentration. Note that in Fig. 2 we show theoretical data, directly as obtained from the DMFT calculation, as well as theory that has been broadened due to lifetime effects. The broadening considered was obtained from the Fermi liquid theory, in which the lifetime decreases quadratically with the binding energy [44] . As is clear from Fig. 2 , both experiment and theory position the Mn-3d states primarily in the valence band of the GaAs host, with the Mn-3d states extending over a broad range of energies. The experimental spectrum has a main peak at ~3.2 eV binding energy, an observation that is captured by theory. Furthermore, the observed broad shoulder, which is located between 4 and 8 eV binding energy, is also well described in the LDA+DMFT excitation spectrum. Overall, the agreement between theory and experiment must be judged as being good. Only in the closest region to the Fermi level can one notice some discrepancies between theory and experiment, where the small peak at ~1 eV binding energy has a slightly high intensity in the calculations, when compared with the observations. 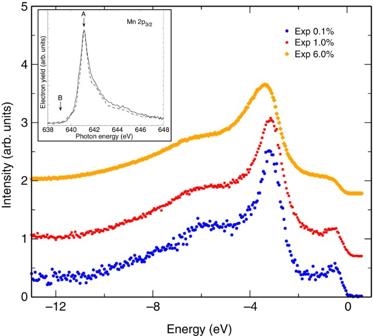Figure 1: Resonant photo-emission spectra of Mn-3d states. Data for various samples of Mn-doped GaAs at different impurities concentration. The 0.1 and 1% spectra are shifted in energy to align with the 6% spectrum at the valence band maximum. In the last case the valence band maximum coincides with the Fermi level. In the inset, the Mn 2p3/2XAS spectra with 0.3 and 6% Mn (dashed and solid lines, respectively) are shown. ‘A’ and ‘B’ indicate the two photon energies used for extracting the resonant photo-emission spectra. Figure 1: Resonant photo-emission spectra of Mn-3d states. Data for various samples of Mn-doped GaAs at different impurities concentration. The 0.1 and 1% spectra are shifted in energy to align with the 6% spectrum at the valence band maximum. In the last case the valence band maximum coincides with the Fermi level. In the inset, the Mn 2p 3/2 XAS spectra with 0.3 and 6% Mn (dashed and solid lines, respectively) are shown. ‘A’ and ‘B’ indicate the two photon energies used for extracting the resonant photo-emission spectra. 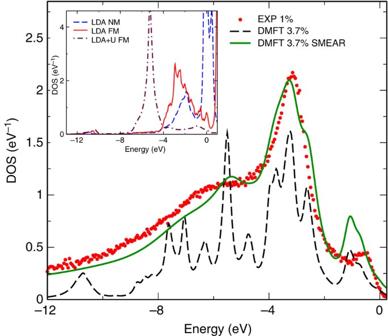Figure 2: Mn-3d PDOS from LDA+DMFT. Resonant photo-emission spectrum of Mn-3d states in Mn-doped GaAs at 1% concentration compared with the Mn-3d projected density of states from LDA+DMFT, with and without Lorentzian smearing. The energy-dependent width of the latter was chosen asτ(ε)=0.04 eV−1×ε2+0.04 eV, to allow a better comparison of the spectral weight with the photo-emission signal. The Fermi level is at zero energy, and no artificial shifts have been applied between theoretical and experimental curves. In the inset, the ferromagnetic (FM) and non-magnetic (NM) LSDA results are shown, together with the LDA+U results. Full size image Figure 2: Mn-3d PDOS from LDA+DMFT. Resonant photo-emission spectrum of Mn-3d states in Mn-doped GaAs at 1% concentration compared with the Mn-3d projected density of states from LDA+DMFT, with and without Lorentzian smearing. The energy-dependent width of the latter was chosen as τ ( ε )=0.04 eV −1 × ε 2 +0.04 eV, to allow a better comparison of the spectral weight with the photo-emission signal. The Fermi level is at zero energy, and no artificial shifts have been applied between theoretical and experimental curves. In the inset, the ferromagnetic (FM) and non-magnetic (NM) LSDA results are shown, together with the LDA+U results. Full size image Host valence band and induced holes In the inset of Fig. 2 , the Mn-3d PDOS for spin-polarized and unpolarized LSDA are reported, and we note that the agreement with the experimental data is less than satisfactory. Focusing on the ferromagnetic LSDA solution, the spectral weight is almost entirely contained in the region with excitation energies below 4 eV, and although the position of the main peak is almost correct, the large shoulder at higher binding energy is totally absent. If electron–electron repulsion is treated in a static Hartree–Fock manner, as for the LDA+U calculations shown in the same inset, the agreement with the experiment does not improve much. The main peak is moved to higher binding energies, its exact position depending on the value of U (refs 35 , 36 , 37 , 38 ), but it is not possible to describe the broad distribution of spectral weight at binding energies between 4 and 8 eV. One must conclude that overall the electronic structure of Mn-doped GaAs is not accurately described by LDA or LDA+U theory, and that dynamical correlation effects have a main role. The experimental results of Gray et al . [30] were in the same study compared with a theory based on LDA. The result is that, despite the sophisticated description of the photo-emission process through the one-step model, theory and experiment do not agree with each other, at least with regard to the spectral features of Mn-3d projected states. The deficiencies of LDA and LDA+U are related to the fact that they are basically single Slater determinant theories, and cannot describe the highly entangled many-body states corresponding to the high spin moment of the half-filled Mn-3d shell and its excited states. This is in line with our recent findings for the transition metals monoxides [45] , where experimental data show a broad distribution of 3d spectral weight not describable within one-particle approximations, but well reproduced by LDA+DMFT. In Fig. 3 , we report the calculated PDOS for the As-4p states, which are the main contributors to the valence band, both for an As atom far away from the Mn impurity and for an As atom close to it. As seen by inspection of the states projected on the As atom far from the Mn impurity, the Fermi level is located at the band edge of the valence band. Looking at the close region around the Fermi level (inset), one sees that the latter is mainly pinned by As-4p states, with a significant contribution of Mn-4p states (not shown). The p-states of the As atom close to the Mn atom show hybridization with the Mn-3d states, which results in spectral features that extend above the Fermi level. As the figure shows, there is a non-negligible distortion of the As-4p states due to the presence of the impurity Mn atom, and this distortion is particularly large close to the Mn impurity. A more quantitative analysis can be made by directly evaluating the hole density for the locally projected bands in LDA+DMFT. For our supercell, the Mn-3d and Mn-4p states contain, respectively, 1 and 3% of the total number of holes, whereas the large majority of holes has As-4p character. The first shell of As nearest neighbours (4 atoms at 0.245 nm) contains 30% of the holes, the second shell (12 atoms at 0.469 nm) 20% and the third shell (6 atoms at 0.616 nm) 21%. The last shell included in the modelling (5 atoms at 0.734 nm) exhibits a sharp drop in the hole density, containing only 7% of the total number of holes. The first shell of Ga nearest neighbours (12 atoms at 0.4 nm) contains 9 and 3% for, respectively, the 4p and 3d states. All the other orbitals contain the remaining holes, without any significant distribution. These numbers point to a local change in the electronic structure located primarily around the impurity and are in close agreement with a recent core level photo-emission study focusing on the Ga-3d spectra from very dilute (Ga,Mn)As (ref. 46 ), where each Mn atom is found to affect a region corresponding to a sphere with 0.7 nm radius. 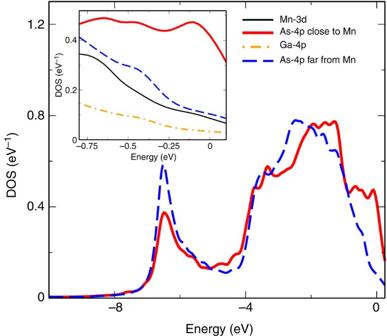Figure 3: As-4p PDOS from LDA+DMFT. LDA+DMFT projected density of states of the As-4p electrons in Mn-doped GaAs, for ions that are close and far from the Mn impurity. The Fermi level is at zero energy. In the inset the projected density of states of the As-4p, the Mn-3d and Ga-4p states are shown in the narrow region around the Fermi level. Figure 3: As-4p PDOS from LDA+DMFT. LDA+DMFT projected density of states of the As-4p electrons in Mn-doped GaAs, for ions that are close and far from the Mn impurity. The Fermi level is at zero energy. In the inset the projected density of states of the As-4p, the Mn-3d and Ga-4p states are shown in the narrow region around the Fermi level. Full size image As shown in Fig. 4 , the precise choice of the parameters describing the Coulomb interaction in the LDA+DMFT calculations does not lead to qualitative differences in the final spectral properties, at least if these changes are limited within a reasonable range of values. As described in the Methods section, the data presented in Figs 2 and 3 are obtained for an average Hubbard parameter U =6 eV and for an average Hund’s exchange parameter J ≃ 1 eV. In the inset of Fig. 4 we show the Mn-3d PDOS in LDA+DMFT for U =5 and U =7 eV. Even for these large changes of U , the main features of the two curves remain similar to that observed in Fig. 2 , and only a small redistribution of spectral weight at high binding energies can be observed. In Fig. 4 , instead, the LDA+DMFT Mn-3d PDOS shown in Fig. 2 , corresponding to U =6 eV and J ≃ 1 eV, is compared with the LDA+DMFT data for U =6 eV and J =0.8 eV. The general features of the spectra are the same, but the two main peaks are shifted towards the Fermi level in the simulation with lower J . From these results, we can see that a change of the parameters in the calculation only slightly modifies the obtained spectrum and does not change the physical picture outlined. 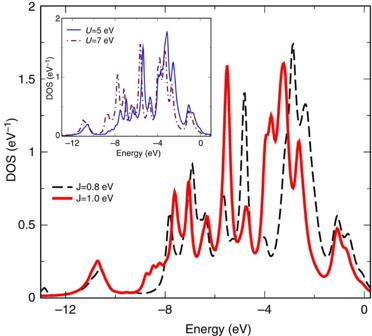Figure 4: Mn-3d PDOS for different parametrizations of the Coulomb interaction. LDA+DMFT projected density of states of the Mn-3d electrons for different values of the exchange parameterJ, andUfixed to 6 eV. In the inset, the same information is shown for different values ofU, withJcalculated from the electron density as described in the main text. The Fermi level is at zero energy. Figure 4: Mn-3d PDOS for different parametrizations of the Coulomb interaction. LDA+DMFT projected density of states of the Mn-3d electrons for different values of the exchange parameter J , and U fixed to 6 eV. In the inset, the same information is shown for different values of U , with J calculated from the electron density as described in the main text. The Fermi level is at zero energy. Full size image The work presented here shows experimental and theoretical photo-emission spectra of bulk Mn-doped GaAs, where good agreement between observations and theory is only found when electron correlations are treated dynamically. To be precise, DMFT in combination with exact diagonalization is shown to reproduce the observed spectral features, whereas other impurity solvers, for example, Hubbard-I (ref. 47 ) or perturbative approaches [48] , are not adequate to this problem (data not shown). A static treatment of electron–electron repulsion, as in LDA+U, is also shown to fail when comparing with experimental spectra. This illustrates that for Mn-doped GaAs, and most probably for DMS materials in general, electronic structure calculations require a more sophisticated treatment than usually found in the literature. On a more detailed level, both our theoretical and experimental results demonstrate the presence of Mn states at the top of the valence band, but that no detached impurity band forms, contrary to what is suggested in the studies by Ohya et al . [28] and Dobrowolska et al . [29] . In addition, we have found that the Mn-3d states contribute very little to the carrier concentration (about 1%). Despite the lack of a detached impurity band, our calculations reveal that the holes have a clear majority of their spectral intensity in the closest shells of As atoms around the Mn impurity, a fact to be taken into consideration when analysing the exchange mechanism of this material. Our results are in very good agreement with recent hard X-ray photo-emission data, which, unlike our study, are obtained by probing directly the ferromagnetic phase [30] . However, the sophisticated photo-emission theory used in that work is still based on the LDA approximation, and therefore suffers of all the inaccuracies mentioned above. Finally, in our theoretical framework, a more quantitative and definite conclusion on the magnetism could probably be obtained by approaching the problem of the evolution of the ordering temperature for different Mn concentrations from first principles. Experiment The photo-emission data were obtained at the Swedish synchrotron radiation facility MAX-lab using the surface end station of the I511 undulator beamline [49] . The samples were prepared in a local molecular beam epitaxy system and were transferred to the photo-emission station in a portable ultrahigh vacuum chamber without being exposed to the atmosphere. The Mn concentrations were determined during growth by means of reflection high-energy electron diffraction oscillations, as described earlier [50] . Survey spectra recorded after transfer showed contamination-free surfaces, and low-energy electron diffraction showed (1 × 2) surface reconstruction. For very low Mn concentration (0.1%), the fractional spots of GaAs(100) c(4 × 4) were still present, but clearly stretched along the ‹100› azimuths, reflecting a transition for (1 × 2) pattern. All spectra presented here were obtained at room temperature from as-grown samples, that is, samples not subjected to postgrowth annealing. After the photo-emission experiment, the magnetic properties were measured ex situ in a SQUID setup. The sample with 6% Mn showed ferromagnetic behaviour below 55 K, whereas none of the other samples showed long-range order above 5 K. Unlike most previous experimental works [50] , [51] , [52] , [53] , the present experiments were carried out on as-grown samples, transferred in ultrahigh vacuum between the growth and analysis systems. This is an essential difference, as the investigated (Ga,Mn)As material is known to be metastable and its surface cannot be reliably restored by traditional preparation methods like Ar sputtering and annealing. Indeed, according to our previous studies [54] , the main Mn-3d emission valence band structure was found significantly closer to the valence band maximum than that reported in all above mentioned reports, and a shift towards higher binding energy was demonstrated to be induced by postgrowth annealing [55] . Although it can be argued that the changes were observed at temperatures above 300 °C, that is, higher than the annealing temperatures applied in the post Ar-sputtering treatments, the energy deposited by the Ar sputtering itself is certainly sufficient to induce structural modifications. By exploiting the momentum selectivity in resonant photo-emission we can focus specifically on the 3d states. As shown, the 3d states are even shallower than suggested by spectra probing the integrated valence band, and the deviation from the value reported in studies by Okabayashi et al . [51] and Rader et al . [52] is even larger. Valence band spectra were recorded at two photon energies, one on the 2p 3/2 absorption peak (A in the inset of Fig. 1 ), the other 2 eV below the peak (B in the inset of Fig. 1 ) and the Mn-3d resonant emission was obtained from the difference between the two spectra. In a previous study [56] , corresponding structures were extracted by combining spectra from (Ga,Mn)As and clean GaAs obtained at the same excitation energy. The main advantage of the procedure adopted here is that it avoids artifacts that inevitably arise due to different surface states on different surfaces. In the extraction of difference spectra it is of course important, particularly in the most dilute cases, that the spectra are properly normalized and aligned in energy. This was accomplished by including the Ga-3d peak in the recorded energy range. By means of this peak the spectra could be aligned with a precision of 1 meV, and the normalization was checked via the absence of any systematic structures in the energy region of Ga-3d emission. For the most dilute cases, it turned out that thermal effects, mainly associated with gradual monochromator heating, had to be taken into account. To minimize these effects, the recording time for each pair of spectra was reduced to about 2 min. To achieve reasonable statistics, a number of difference spectra (typically 50–100) were added after proper alignment. In contrast to the recently published hard X-ray photo-emission from (Ga,Mn)As (ref. 30 ), the present data are quite surface-sensitive due to the relatively short electron mean free path (around 1.5 nm). However, due to the rapidly falling Mn-3d/As-4p cross-section ratio with increasing photon energy [57] the emission from Mn-3d in the study by Gray et al . [30] is hardly discernible. In contrast, under the resonant conditions used here, the Mn-3d emission is enhanced selectively and dominates the spectrum for samples with Mn concentrations above 1%. Theory The theoretical spectra have been calculated by means of an LDA+DMFT technique [58] , [59] based on a full-potential linear-muffin tin orbital method [60] , which is particularly suitable for large supercell geometries. The Mn-doped GaAs was modelled with a supercell Ga 26 MnAs 27 , corresponding to a Mn concentration of 3.7%. The experimental lattice constant a =10.681 a.u. was used, and the Brillouin zone was sampled with a mesh of 256 k-points. The LDA+DMFT scheme was applied to explicitly treat the local Coulomb interaction between the localized Mn-3d electrons. The 4-index rotationally invariant Coulomb interaction matrix was generated from the Slater parameters F 0 , F 2 and F 4 . The choice of the average Coulomb repulsion F 0 , which corresponds to the Hubbard U, is rather problematic, as no calculations based on constrained LDA or random phase approximation (RPA) methods are found in the literature. Therefore, we have considered values between 4 and 7 eV, which are the accepted strengths of the Coulomb repulsion for bulk metallic γ-Mn (ref. 48 ) and MnO (ref. 45 ). The main results of the paper are presented for the intermediate value U =6 eV, whereas results for smaller and larger values are discussed at the end of the Results section. F 2 and F 4 are easier to evaluate and therefore were calculated directly from the electronic density as done in the study by Thunström et al . [45] . The calculated values correspond to the average Hund’s exchange parameter J ≃ 1 eV. The LDA+DMFT results for J =0.8 eV, shown in Fig. 4 , were based on F 2 and F 4 obtained by means of fixed atomic ratios [41] , [42] . The effective impurity problem arising in LDA+DMFT has been solved through exact diagonalization method, as described in the study by Thunström et al . [45] The fermionic bath interacting with the atomic impurity has been approximated by means of 22 auxiliary bath spin-orbitals: 18 bath states were coupled to the strongly hybridizing Mn t 2g states, whereas only 4 bath states were coupled to the weakly hybridizing Mn e g states. All the calculations have been made for the paramagnetic phase at T =400 K and using 1,200 fermionic Matsubara frequencies, and double-counting problem has been considered in the fully localized limit [41] , [42] . Finally, in the calculation of the hole densities, we have considered only the atoms included in one supercell and their multiplicity, consistently with our physical modelling and previous literature [38] . How to cite this article: Di Marco, I. et al . Electron correlations in Mn x Ga 1– x As as seen by resonant electron spectroscopy and dynamical mean field theory. Nat. Commun. 4:2645 doi: 10.1038/ncomms3645 (2013).